Oxytocin is an age-specific circulating hormone that is necessary for muscle maintenance and regeneration The regenerative capacity of skeletal muscle declines with age. Previous studies suggest that this process can be reversed by exposure to young circulation; however, systemic age-specific factors responsible for this phenomenon are largely unknown. Here we report that oxytocin—a hormone best known for its role in lactation, parturition and social behaviours—is required for proper muscle tissue regeneration and homeostasis, and that plasma levels of oxytocin decline with age. Inhibition of oxytocin signalling in young animals reduces muscle regeneration, whereas systemic administration of oxytocin rapidly improves muscle regeneration by enhancing aged muscle stem cell activation/proliferation through activation of the MAPK/ERK signalling pathway. We further show that the genetic lack of oxytocin does not cause a developmental defect in muscle but instead leads to premature sarcopenia. Considering that oxytocin is an FDA-approved drug, this work reveals a potential novel and safe way to combat or prevent skeletal muscle ageing. The proportion of people over the age of 60 is growing faster than any other age group, as a result of both longer life expectancy and declining fertility rates, thus enhancing the quality of life as people age is of major importance. With ageing, the capacity of our tissues to maintain homeostasis and regenerate declines and eventually fails, leading to degenerative disorders and eventual organ failure. The reduction in muscle mass in humans starts in the third decade of life and accelerates after the fifth decade, resulting in a decrease in strength and agility [1] . Muscle ageing is characterized by a deficiency in muscle regeneration after injury and by muscle atrophy associated with altered muscle function, defined as sarcopenia [2] . The limiting step in muscle regeneration after injury is the activation of the muscle stem cells, or satellite cells. They need to break quiescence and proliferate in order to form new myofibres or fuse with damaged ones. Satellite cells from old muscle are intrinsically able to repair damaged muscle, but are reversibly inhibited by the aged niche, yet can be quickly rescued for productive tissue repair by a number of experimental methods, including heterochronic parabiosis [3] . While the rejuvenating effects of heterochronic parabiosis have been observed in several tissues such as muscle, brain, liver, pancreas and heart [4] , [5] , [6] , [7] , [8] , [9] , the molecular mechanisms are not fully understood and only a few potential systemic factors responsible for this phenomena have been identified. A few pro-ageing circulating factors that increase in old animals have been identified, including transforming growth factor (TGF)-β and Wnt signalling pathway effectors, which are deleterious for muscle regeneration [5] , [10] , as well as the CCL11 chemokine that leads to impaired neurogenesis and decreased cognition and memory [6] . To date, few circulating molecules decreasing with age have been identified to be responsible for skeletal muscle ageing. Considering that oxytocin (OT) levels decrease after ovariectomy, which mimics hormonal ageing [11] , and that myoblasts express the OT receptor (OTR) [12] , we hypothesized that OT might be among the key circulating age-specific determinants of maintenance and repair of skeletal muscle. OT is a nonapeptide mainly produced by the hypothalamus and stored in the neurohypophysis. It acts via its receptor both centrally as a neuromodulator and peripherally as a hormone, released by the neurohypophysis into the circulation. The OTR is a class I G-protein-coupled receptor, which upon OT binding activates protein kinase C and induces intracellular calcium release that acts as a second messenger to induce a cascade of intracellular changes and activity [13] . OT is best known for its role in lactation and parturition [14] as well as in social behaviours, promoting trust and bonding [15] . While the role of OT in supporting tissue homeostasis and regeneration is poorly documented, recent published work proposed a role of OT in preventing osteoporosis and obesity [11] , [16] , [17] , [18] , [19] , [20] and in improving myocardium recovery after ischaemic injury [21] . In addition, OT has been shown to facilitate in vitro differentiation of mesenchymal stem cells towards cardiomyogenesis and osteogenesis and to inhibit adipocyte differentiation [11] , [22] . Here we show that plasma levels of OT and the levels of OTR in muscle stem cells dramatically decline with age and demonstrate that OT is required for skeletal muscle tissue regeneration and homeostatic maintenance. Importantly, we show that short-term systemic OT delivery restores muscle regeneration in old mice by improving aged muscle stem cell function, while pharmacologic attenuation of OT signalling with a selective antagonist alters muscle regeneration in young mice. Confirming the dependence of muscle maintenance and repair on OT, mice deficient for Ot present signs of premature muscle tissue ageing: defective muscle regeneration and a decrease in muscle mass and fibre size characteristic of sarcopenia at only 12 months of age. Our results suggest that OT per se or deliberate modulation of OT signalling could become a potential treatment to combat the age-related decline in muscle tissue maintenance and repair. Systemic OT and OTR levels in satellite cells decline with age Since circulating OT levels decrease after ovariectomy, which mimics hormonal ageing [11] , we hypothesized that its level would decrease during natural ageing. OT plasma levels were measured in young (2- to 4-month-old) and old (18- to 24-month-old) C57/BL6 male mice, using an OT-specific enzyme immunoassay. A significant threefold decrease was observed in aged mice as compared with young, suggesting that endocrine levels of OT decline with age ( Fig. 1a ). Little is known about the expression of the OTR in skeletal muscle either in general or in an age-specific way; thus, we examined OTR protein expression in young and old skeletal muscle. Western blotting analysis demonstrates that OTR is detected in whole skeletal muscle ( Fig. 1b ). Similar levels of OTR were observed in young and old whole muscle lysates that contain, in addition to proteins from muscle fibres and satellite cells, proteins from other cell types including vascular and immune cells, adipocytes and fibroblasts ( Fig. 1b,d ). Notably, when protein lysates were prepared from muscle stem cells, OTR was found to be expressed at significantly higher levels in young satellite cells as compared with old ( Fig. 1c,e ). These results demonstrate that with ageing the decline in the circulating OT hormone is compounded by diminished levels of OTR in the old muscle stem cells. Confirming the western blotting data, immunofluorescence analysis of muscle tissue sections revealed that OTR was indeed expressed in cells that were observed in the satellite cell position ( Fig. 1f , top) and colocalized with the satellite cell marker Pax7 in quiescent and injury-activated satellite cells ( Fig. 1f , middle panels). Although most Pax7-positive satellite cells express OTR, expression of this receptor was also observed in many Pax7-negative cells ( Fig. 1f ), suggesting that OT acts on several cell types in skeletal muscle. 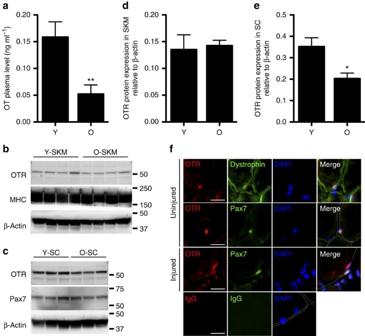Figure 1: Systemic oxytocin declines with age and oxytocin receptor is expressed in skeletal muscle satellite cells. (a) OT plasmatic levels were quantified using enzyme immunoassay in young (2- to 4-month-old) and aged (18- to 24-month-old) C57BL/6 male mice. Data represent mean±s.e.m. (n=6 young versusn=7 old). Two-tailed unpaired Student’st-test, **Pvalue <0.01. (b,c) Whole skeletal muscle (gastrocnemius) protein extracts (b), and hind limb satellite cell protein extracts (c) were prepared from young and old non-injured mice. OTR, Pax7 and myosin heavy chain (MHC) were assayed using western blot analysis. Thirty micrograms of protein were loaded per lane and β-actin was used as a loading control. Inb,c, Y-SKM: young skeletal muscle; O-SKM: old skeletal muscle; Y-SC: young satellite cell; O-SC: old satellite cell. (d,e) Quantification of western blot fromb,c, using the Image J software. Data represent mean±s.e.m. (n=4 Y-SKM,n=4 O-SKM,n=3 Y-SC andn=3 O-SC). Two-tailed unpaired Student’st-test, *Pvalue <0.05. (f) Cross-sections from non-injured and 3-day-injured tibialis anterior muscle were immunostained for OTR and dystrophin or OTR and Pax7, as indicated, and counterstained with DAPI. IgG control are displayed (bottom) and dashed lines delineate muscle fibres. Scale bars represent 20 μm. Figure 1: Systemic oxytocin declines with age and oxytocin receptor is expressed in skeletal muscle satellite cells. ( a ) OT plasmatic levels were quantified using enzyme immunoassay in young (2- to 4-month-old) and aged (18- to 24-month-old) C57BL/6 male mice. Data represent mean±s.e.m. ( n =6 young versus n =7 old). Two-tailed unpaired Student’s t -test, ** P value <0.01. ( b , c ) Whole skeletal muscle (gastrocnemius) protein extracts ( b ), and hind limb satellite cell protein extracts ( c ) were prepared from young and old non-injured mice. OTR, Pax7 and myosin heavy chain (MHC) were assayed using western blot analysis. Thirty micrograms of protein were loaded per lane and β-actin was used as a loading control. In b , c , Y-SKM: young skeletal muscle; O-SKM: old skeletal muscle; Y-SC: young satellite cell; O-SC: old satellite cell. ( d , e ) Quantification of western blot from b , c , using the Image J software. Data represent mean±s.e.m. ( n =4 Y-SKM, n =4 O-SKM, n =3 Y-SC and n =3 O-SC). Two-tailed unpaired Student’s t -test, * P value <0.05. ( f ) Cross-sections from non-injured and 3-day-injured tibialis anterior muscle were immunostained for OTR and dystrophin or OTR and Pax7, as indicated, and counterstained with DAPI. IgG control are displayed (bottom) and dashed lines delineate muscle fibres. Scale bars represent 20 μm. Full size image Systemic decline in OT causes poor regeneration of old muscle To determine whether the age-specific decrease in systemic OT is responsible for the decline in muscle regeneration that is typical of old mice, we systemically administered OT to old mice and an OT-selective antagonist (OTA) to young mice and studied the success in muscle regeneration after cardiotoxin-induced injury. The schematic for this study is shown in Fig. 2a . Five days post injury, robust muscle regeneration was observed in young mice, based on the high numbers of newly formed (eMyHC+) fibres with centrally located nuclei in the injured area ( Fig. 2b,c ). As expected, a significant decline in the formation of new muscle fibres was evident in old mice. Interestingly, subcutaneous injections of OT improved muscle regeneration in the old mice to a level comparable to the young. In young mice, in which muscle regeneration occurs efficiently, ectopic OT had no effect ( Fig. 2b,c ). Importantly, a significant decrease in muscle regeneration, to a level similar to that seen in old mice, ensued when young mice were administered with OTA ( Fig. 2b,c ). 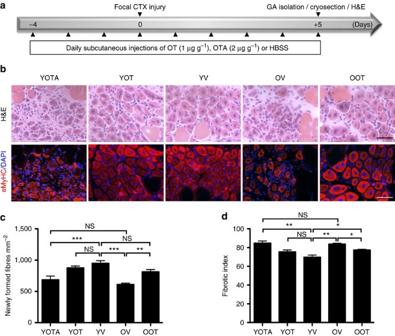Figure 2: Age-specific systemic oxytocin decline plays a key role in the defective muscle regeneration observed upon ageing. (a) Schematic of the experimental procedure. Cardiotoxin (CTX) muscle injury was performed on day 0. Four days before muscle injury and over the course of the experiment, mice were administered OT (1 μg g−1of mice), OTA (2 μg g−1of mice) or vehicle (HBSS) daily. Five days after muscle injury, mice were euthanized and gastrocnemius (GA) muscles were dissected. Cross-sections (10 μm) were stained for haematoxylin and eosin (H&E). (b) H&E (top) and eMyHC (bottom) staining of cardiotoxin-injured GA muscle cross-sections from mice injected with OT, OTA or vehicle (HBSS). Scale bars represent 50 μm. (c) Muscle regeneration was quantified by scoring the number of newly formed fibres (eMyHC-positive fibres with centrally located nuclei) in the injured area of GA cross-sections. Data represent mean±s.e.m. (n=9 YV,n=5 OV,n=6 YOT,n=6 OOT,n=5 YOTA). One-way analysis of variance (ANOVA) withpost hocNewman–Keuls test, **Pvalue <0.01, ***Pvalue <0.001, NS: not significant. (d) Fibrosis quantification of GA muscle cross-sections 5 days after injury. The fibrotic index represents the percentage of the injury area occupied by connective tissue. Data represent mean±s.e.m. (n=3 YV,n=3 OV,n=3 YOT,n=3 OOT,n=3 YOTA). One-way ANOVA withpost hocNewman–Keuls test, *Pvalue <0.05, **Pvalue <0.01, NS: not significant. Inb–d, YOTA: young injected with OTA; YOT: young injected with OT; YV: young injected with vehicle, OV: old injected with vehicle; OOT: old injected with OT. Figure 2: Age-specific systemic oxytocin decline plays a key role in the defective muscle regeneration observed upon ageing. ( a ) Schematic of the experimental procedure. Cardiotoxin (CTX) muscle injury was performed on day 0. Four days before muscle injury and over the course of the experiment, mice were administered OT (1 μg g −1 of mice), OTA (2 μg g −1 of mice) or vehicle (HBSS) daily. Five days after muscle injury, mice were euthanized and gastrocnemius (GA) muscles were dissected. Cross-sections (10 μm) were stained for haematoxylin and eosin (H&E). ( b ) H&E (top) and eMyHC (bottom) staining of cardiotoxin-injured GA muscle cross-sections from mice injected with OT, OTA or vehicle (HBSS). Scale bars represent 50 μm. ( c ) Muscle regeneration was quantified by scoring the number of newly formed fibres (eMyHC-positive fibres with centrally located nuclei) in the injured area of GA cross-sections. Data represent mean±s.e.m. ( n =9 YV, n =5 OV, n =6 YOT, n =6 OOT, n =5 YOTA). One-way analysis of variance (ANOVA) with post hoc Newman–Keuls test, ** P value <0.01, *** P value <0.001, NS: not significant. ( d ) Fibrosis quantification of GA muscle cross-sections 5 days after injury. The fibrotic index represents the percentage of the injury area occupied by connective tissue. Data represent mean±s.e.m. ( n =3 YV, n =3 OV, n =3 YOT, n =3 OOT, n =3 YOTA). One-way ANOVA with post hoc Newman–Keuls test, * P value <0.05, ** P value <0.01, NS: not significant. In b – d , YOTA: young injected with OTA; YOT: young injected with OT; YV: young injected with vehicle, OV: old injected with vehicle; OOT: old injected with OT. Full size image The deficiency in skeletal muscle regeneration observed in aged mice is associated with an increase in fibrotic tissue formation [5] , [23] . As expected, the fibrotic index was greater in old mice as compared with young ( Fig. 2d and Supplementary Fig. 1a ). Ectopic OT significantly decreased the fibrotic index in old mice, whereas OTA injections increased fibrosis in young mice ( Fig. 2d and Supplementary Fig. 1a ). These data demonstrate that one consequence of the age-specific systemic decline in OT is poor regeneration of skeletal muscle accompanied by increased fibrosis. Importantly, ectopic OT rapidly rescued repair of damaged old muscle, while OTA quickly incapacitated the regeneration of young muscle. OT mediates the regenerative potential of muscle stem cells Satellite cell activation/proliferation are the main limiting steps in old muscle regeneration. Exposure to a young environment has been shown to restore muscle regeneration by promoting satellite cell proliferation [3] , [4] , [24] . Since ectopic OT exposure over a short period of time rescued the repair of damaged old muscle, we evaluated whether the decreased level of OT in old was responsible for the lack of satellite cell proliferation in vivo . OT was administered to old mice daily starting 6 days before cardiotoxin-induced muscle injury ( Fig. 3a ). To monitor cell division in vivo , BrdU was injected subcutaneously 12 h before mice were euthanized. Three days after injury, tibialis anterior (TA) muscles were isolated, and the percentages of BrdU and Desmin double-positive cells (that is, proliferating myogenic progenitor cells that were generated by satellite cells activated in response to tissue injury) were quantified in the injury area in muscle sections ( Fig. 3b,c ). As we have previously published, these myogenic cells co-express Pax7 and Desmin, while the non-myogenic Desmin-positive cells represent less than 2% in such experiments [25] , [26] . A threefold decrease in myogenic cell proliferation was observed in old muscles as compared with young ( Fig. 3c ). Importantly and in agreement with the rescue of muscle repair, ectopic OT significantly improved myogenic cell proliferation in vivo ( Fig. 3c ). 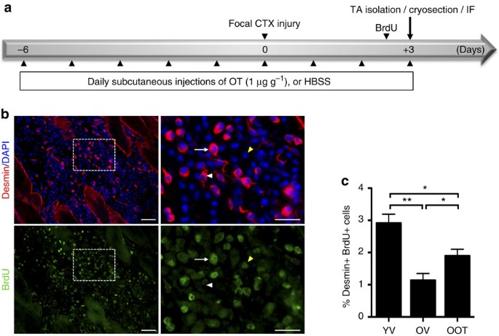Figure 3: Oxytocin improves muscle stem cell proliferationin vivoafter injury. (a) Schematic of the experimental procedure. Cardiotoxin (CTX) muscle injury was performed on day 0. Six days before muscle injury and over the course of the experiment, mice were administered OT (1 μg g−1of mice) or vehicle (HBSS) daily. Twelve hours before they were euthanized, mice were administered with BrdU (50 μg g−1of mice, IP). Three days after muscle injury, TA muscles were isolated. (b) Representative micrographs of 3-day-injured TA muscle cross-sections (10 μm) immunostained for BrdU and Desmin and counterstained with DAPI. Right panels represent magnifications of the dashed area from left panels. White arrow indicates a BrdU and Desmin double-positive cell, yellow and white arrowheads indicate BrdU or Desmin single-positive cells, respectively. Scale bars represent 100 μm (left panels) and 50 μm (right panels). (c) Quantification of the percentage of proliferating myogenic cells (Desmin+ and BrdU+). Data represent mean±s.e.m. (n=4 YV,n=4 OV,n=4 OOT), one-way ANOVA withpost hocNewman–Keuls test, *Pvalue <0.05, **Pvalue <0.01. Figure 3: Oxytocin improves muscle stem cell proliferation in vivo after injury. ( a ) Schematic of the experimental procedure. Cardiotoxin (CTX) muscle injury was performed on day 0. Six days before muscle injury and over the course of the experiment, mice were administered OT (1 μg g −1 of mice) or vehicle (HBSS) daily. Twelve hours before they were euthanized, mice were administered with BrdU (50 μg g −1 of mice, IP). Three days after muscle injury, TA muscles were isolated. ( b ) Representative micrographs of 3-day-injured TA muscle cross-sections (10 μm) immunostained for BrdU and Desmin and counterstained with DAPI. Right panels represent magnifications of the dashed area from left panels. White arrow indicates a BrdU and Desmin double-positive cell, yellow and white arrowheads indicate BrdU or Desmin single-positive cells, respectively. Scale bars represent 100 μm (left panels) and 50 μm (right panels). ( c ) Quantification of the percentage of proliferating myogenic cells (Desmin+ and BrdU+). Data represent mean±s.e.m. ( n =4 YV, n =4 OV, n =4 OOT), one-way ANOVA with post hoc Newman–Keuls test, * P value <0.05, ** P value <0.01. Full size image To further study the effect of OT on satellite cell proliferation and differentiation, we performed an ex vivo analysis, as described in the schematic of Fig. 4a . Three days post injury, muscles were isolated and digested into bulk myofibres as previously described [25] , [27] and cells were cultured in their own mouse’s respective serum for 24 h ( Fig. 4a ). In order to label the cells that were activated in vivo in response to muscle injury, BrdU was injected subcutaneously 12 h before mice were euthanized. Myogenic proliferation of cells activated in vivo was quantified by calculating the percentage of BrdU and Desmin double-positive cells, which as mentioned above is a sensitive and accurate way to measure the age-specific differences in myogenicity [24] , [25] , [27] . A 41% decrease in proliferation was observed in the old activated satellite cells as compared with young ( Fig. 4b, c ). Confirming the in vivo data observed in Fig. 3c , ectopic OT restored the myogenic proliferation of old satellite cells to a level comparable to young. Moreover, decreased myogenic proliferation was observed when young mice were treated with OTA ( Fig. 4b,c ). We also observed that the proliferation of activated satellite cells derived from young mice administered with OT tended to increase. 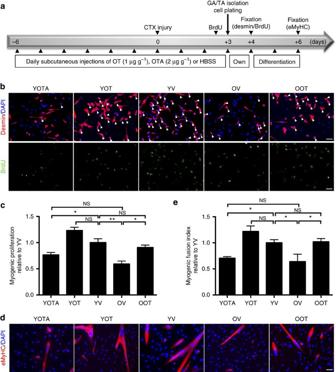Figure 4: Oxytocin rejuvenates muscle stem cell function in injured tissue. (a) Schematic of the experimental procedure. Cardiotoxin (CTX) muscle injury was performed on day 0. Six days before muscle injury and over the course of the experiment, mice were administered OT (1 μg g−1of mice), OTA (2 μg g−1of mice) or vehicle (HBSS) daily. Twelve hours before they were euthanized, mice were administered with BrdU (50 μg g−1of mice, IP). Three days after muscle injury, gastrocnemius (GA) and tibialis anterior (TA) muscles were isolated and digested into bulk fibres. Cells were cultured in their mouse’s respective sera (shortened as ‘own’ on the schematic) for 24 h and either fixed and stained for Desmin and BrdU or induced to differentiate for 48 h and subsequently fixed and stained for eMyHC. (b,c) Myogenic cell proliferation. Muscle fibre-associated activated satellite cells were isolated 3 days after injury from mice injected with OT, OTA or vehicle (HBSS), plated in media containing their mouse’s respective sera and fixed 24 h after plating. (b) Representative micrographs of cells immunostained for Desmin and BrdU and counterstained with DAPI. Scale bars represent 50 μm. (c) Quantification of the percentage of proliferating myogenic cells (Desmin+ and BrdU+). Data represent mean±s.e.m. (n=6 YV,n=3 OV,n=3 YOT,n=3 OOT,n=5 YOTA). (d,e) Myogenic fusion index. Muscle fibre-associated activated satellite cells were isolated 3 days after injury from mice injected with OT, OTA or vehicle (HBSS) and plated in media containing their mouse’s respective sera for 24 h. Cells were then induced to differentiate in mitogen-low fusion medium for 48 h, fixed and immunostained for eMyHC using DAPI to label all nuclei. (d) Representative micrographs. Scale bar represents 50 μm. (e) Quantification of the percentage of nuclei in eMyHC+ myotubes. Data represent mean±s.e.m. (n=8 YV,n=5 OV,n=6 YOT,n=6 OOT,n=5 YOTA). Inb–eYOTA: young injected with OTA; YOT: young injected with OT; YV: young injected with vehicle, OV: old injected with vehicle; OOT: old injected with OT. One-way ANOVA withpost hocNewman–Keuls test, *Pvalue<0.05, **Pvalue<0.01, ***Pvalue<0.001, NS: not significant. Figure 4: Oxytocin rejuvenates muscle stem cell function in injured tissue. ( a ) Schematic of the experimental procedure. Cardiotoxin (CTX) muscle injury was performed on day 0. Six days before muscle injury and over the course of the experiment, mice were administered OT (1 μg g −1 of mice), OTA (2 μg g −1 of mice) or vehicle (HBSS) daily. Twelve hours before they were euthanized, mice were administered with BrdU (50 μg g −1 of mice, IP). Three days after muscle injury, gastrocnemius (GA) and tibialis anterior (TA) muscles were isolated and digested into bulk fibres. Cells were cultured in their mouse’s respective sera (shortened as ‘own’ on the schematic) for 24 h and either fixed and stained for Desmin and BrdU or induced to differentiate for 48 h and subsequently fixed and stained for eMyHC. ( b , c ) Myogenic cell proliferation. Muscle fibre-associated activated satellite cells were isolated 3 days after injury from mice injected with OT, OTA or vehicle (HBSS), plated in media containing their mouse’s respective sera and fixed 24 h after plating. ( b ) Representative micrographs of cells immunostained for Desmin and BrdU and counterstained with DAPI. Scale bars represent 50 μm. ( c ) Quantification of the percentage of proliferating myogenic cells (Desmin+ and BrdU+). Data represent mean±s.e.m. ( n =6 YV, n =3 OV, n =3 YOT, n =3 OOT, n =5 YOTA). ( d , e ) Myogenic fusion index. Muscle fibre-associated activated satellite cells were isolated 3 days after injury from mice injected with OT, OTA or vehicle (HBSS) and plated in media containing their mouse’s respective sera for 24 h. Cells were then induced to differentiate in mitogen-low fusion medium for 48 h, fixed and immunostained for eMyHC using DAPI to label all nuclei. ( d ) Representative micrographs. Scale bar represents 50 μm. ( e ) Quantification of the percentage of nuclei in eMyHC+ myotubes. Data represent mean±s.e.m. ( n =8 YV, n =5 OV, n =6 YOT, n =6 OOT, n =5 YOTA). In b – e YOTA: young injected with OTA; YOT: young injected with OT; YV: young injected with vehicle, OV: old injected with vehicle; OOT: old injected with OT. One-way ANOVA with post hoc Newman–Keuls test, * P value<0.05, ** P value<0.01, *** P value<0.001, NS: not significant. Full size image To study whether these Brdu and Desmin double-positive satellite cell progeny were functionally competent, we evaluated their myogenic differentiation potential. As illustrated in Fig. 4a , cells isolated from muscles at 3 days post injury were cultured for 24 h in their mouse’s respective serum and were switched to differentiation medium for 48 h, when a pronounced age-specific decline in generation of de novo myotubes is typically detected. The myogenic fusion index (the number of nuclei included in de novo formed eMyHC+ myotubes as a fraction of the total nuclei) was then scored to assess cell differentiation. Supporting the observed increase in the number of newly regenerated eMyHC+ fibres in vivo after OT injection ( Fig. 2b,c ), systemic administration of OT to old mice rejuvenated the myofibre-forming capacity of satellite cells responding to tissue injury ( Fig. 4d,e ). In agreement with the idea that OT is required for myogenicity, when OT signalling was antagonized in young mice not only the proliferation but also the differentiation declined to levels similar to those of old animals, with their low circulatory OT ( Fig. 4d,e ). These results demonstrate that myogenic proliferation and subsequent differentiation depend on ‘youthful’ levels of OT. Since we showed that OTR was expressed in skeletal muscle satellite cells ( Fig. 1c,e,f ), we hypothesized that OT acts directly on myogenic cells. To test this hypothesis, satellite cells were freshly isolated from cardiotoxin-injured muscles and plated in medium containing their own mouse serum supplemented or not with OT for 24 h. As previously published [28] and shown in Supplementary Fig. 2 , satellite cell purity was similar for young and old cells and greater than 90%. OT increased the proliferative capacity of old satellite cells cultured in old serum to similar levels of young cells cultured in young serum, as shown by the increased percentage of Ki67-positive activated muscle stem cells and the diminished expression of the cyclin-dependent kinase inhibitor 1, p21 ( Fig. 5a–c ). No effects of OT were observed on young satellite cells, in agreement with the higher levels of endogenous OT in young circulation ( Fig. 1a ). OT also promoted the proliferation of primary myogenic progenitors as shown by a threefold increase in the percentage of BrdU-positive cells ( Fig. 5d, e ). 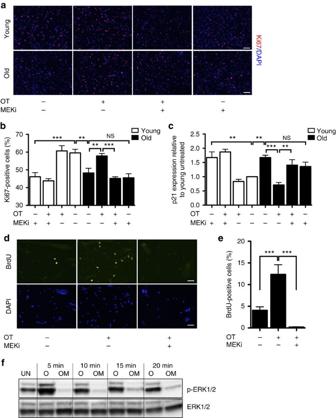Figure 5: Oxytocin improves myogenic progenitor cell proliferation via activation of the MAPK/ERK pathway. (a,b) Activated satellite cells were isolated 3 days after injury from young or old mice, cultured for 24 h in media containing their own mouse’s respective sera supplemented with OT (30 nM), PD98059 MEK inhibitor (50 μM) or OT plus MEK inhibitor, fixed and stained for Ki67 and counterstained for DAPI. (a) Representative micrographs. Scale bars represent 200 μm. (b) Quantification of the percentage of proliferating (Ki67+) satellite cells. Data represent mean±s.e.m. (n=4 mice per group). Two-way ANOVA withpost hocBonferroni test, **Pvalue <0.01, ***Pvalue <0.001, NS: not significant. (c) p21 mRNA relative expression analysed with qRT–PCR. RNA was extracted from satellite cells isolated and cultured as ina. GAPDH was used as reference gene (n=3 mice per group). Two-way ANOVA withpost hocBonferroni test, **Pvalue <0.01, ***Pvalue <0.001, NS: not significant. (d,e) Primary myogenic progenitors were cultured in the presence or absence of OT (30 nM), and UO126 MEK inhibitor (10 μM) for 48 h. BrdU was added to the culture medium during the last hour. Cells were then fixed, immunostained for BrdU and counterstained with DAPI. (d) Representative micrographs. Scale bars represent 50 μm. (e) The percentages of BrdU-positive cells were scored. Data represent mean±s.e.m. (n=8 independent experiments performed on different primary cultures). One-way ANOVA withpost hocNewman–Keuls test, ***Pvalue <0.001, NS: not significant. (f) Primary myogenic progenitors were serum-starved overnight and then treated with OT (30 nM) or OT (30 nM) plus UO126 MEK inhibitor (10 μM) for up to 20 min. ERK1/2 and phospho-ERK1/2 were assayed with western blot analysis. O: OT, OM: OT plus UO126 MEK inhibitor, UN: untreated. Figure 5: Oxytocin improves myogenic progenitor cell proliferation via activation of the MAPK/ERK pathway. ( a , b ) Activated satellite cells were isolated 3 days after injury from young or old mice, cultured for 24 h in media containing their own mouse’s respective sera supplemented with OT (30 nM), PD98059 MEK inhibitor (50 μM) or OT plus MEK inhibitor, fixed and stained for Ki67 and counterstained for DAPI. ( a ) Representative micrographs. Scale bars represent 200 μm. ( b ) Quantification of the percentage of proliferating (Ki67+) satellite cells. Data represent mean±s.e.m. ( n =4 mice per group). Two-way ANOVA with post hoc Bonferroni test, ** P value <0.01, *** P value <0.001, NS: not significant. ( c ) p21 mRNA relative expression analysed with qRT–PCR. RNA was extracted from satellite cells isolated and cultured as in a . GAPDH was used as reference gene ( n =3 mice per group). Two-way ANOVA with post hoc Bonferroni test, ** P value <0.01, *** P value <0.001, NS: not significant. ( d , e ) Primary myogenic progenitors were cultured in the presence or absence of OT (30 nM), and UO126 MEK inhibitor (10 μM) for 48 h. BrdU was added to the culture medium during the last hour. Cells were then fixed, immunostained for BrdU and counterstained with DAPI. ( d ) Representative micrographs. Scale bars represent 50 μm. ( e ) The percentages of BrdU-positive cells were scored. Data represent mean±s.e.m. ( n =8 independent experiments performed on different primary cultures). One-way ANOVA with post hoc Newman–Keuls test, *** P value <0.001, NS: not significant. ( f ) Primary myogenic progenitors were serum-starved overnight and then treated with OT (30 nM) or OT (30 nM) plus UO126 MEK inhibitor (10 μM) for up to 20 min. ERK1/2 and phospho-ERK1/2 were assayed with western blot analysis. O: OT, OM: OT plus UO126 MEK inhibitor, UN: untreated. Full size image OT directly acts in satellite cells via the MAPK/ERK pathway Since the mitogen-activated protein kinase (MAPK) signalling pathway plays an important role in muscle stem cell activation/proliferation [29] , [30] , [31] , [32] , [33] , [34] and phospho-ERK1/2 is a well-documented downstream effector of OT in other cell types [11] , [35] , we postulated that OT could be a physiological inducer of MAPK that promotes myogenic cell proliferation via the phosphorylation of ERK1/2. Indeed, addition of a MEK inhibitor (MEKi) decreased the proliferation of young satellite cells and increased the expression of p21 to old levels ( Fig. 5a–c ). In accordance with the idea that OT signals via MAPK in supporting adult myogenesis, the effects of ectopic OT on freshly isolated activated satellite cells and on primary myogenic progenitor cells were abolished in the presence of MEKi ( Fig. 5a–e ). To confirm the ability of OT to induce ERK1/2 phosphorylation, primary myogenic progenitor cells were stimulated for 5–20 min with OT in the presence or absence of MEKi. ERK1/2 phosphorylation was greatly induced 5 min after stimulation with OT ( Fig. 5f ). At 10 min ERK1/2 phosphorylation started to decrease and returned to the basal level by 20 min ( Fig. 5f ). In support of functional effects of OT on myogenic cell proliferation shown above, MEKi prevented OT-induced ERK1/2 phosphorylation, reducing the levels of phospho-ERK1/2 below the basal level observed in untreated cells ( Fig. 5f ), all confirming activation of the MAPK pathway by its endogenous ligand for productive myogenic responses. Ot -deficient mice display premature muscle ageing To confirm these findings in a genetic model, we studied muscle regeneration after cardiotoxin-induced injury in Ot knockout (KO) mice (B6;129S-Oxttm1Wsy/J). As compared with their wild-type (WT) littermates, we observed a progressive decline in muscle regeneration of Ot KO mice that was noticeable at 3 months of age and became pronounced and significant at 12 months of age ( Fig. 6a,b ). The decline in muscle regeneration observed between 1-year-old WT and Ot KO mice is comparable to the one measured between young (2- to 4-month-old) and old (18- to 24-month-old) WT C57/BL6 mice. In accordance with the data on the in vivo decline in the myogenic cell proliferation in old C57/BL6 mice, a decrease in activated satellite cell proliferation was observed in Ot KO mice when compared with WT littermates ( Fig. 6c ). A significant decline in muscle maintenance and repair is not expected and was not observed in WT mice at 12 months of age ( Fig. 6b ); thus, it is very interesting that the lack of OT prematurely ages the animals in this aspect. 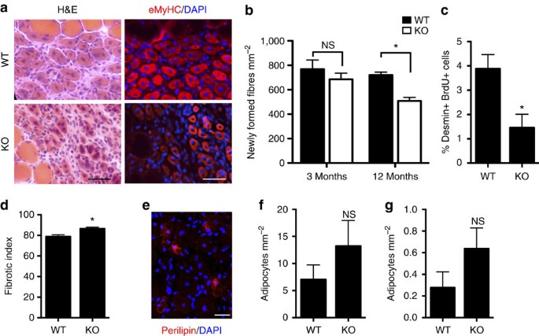Figure 6: Impaired muscle regeneration in mice lacking oxytocin. (a) H&E (top) and eMyHC (bottom) of cardiotoxin-injured gastrocnemius (GA) muscle cross-sections from 12-month-old WT andOtKO mice. Scale bars represent 50 μm. (b) Muscle regeneration quantification of 3- and 12-month-old WT orOtKO mice was performed by scoring the number of newly formed fibres (eMyHC-positive fibres with centrally located nuclei) in the injured area of GA cross-sections. Data represent mean±s.e.m. (n=6 WT andn=4 KO for the 3-month-old mice,n=4 WT andn=5 KO for the 12-month-old). Two-way ANOVA withpost hocBonferroni test, *Pvalue <0.05, NS: not significant. (c) Quantification of the percentage of proliferating myogenic cells (Desmin+ and BrdU+) of 3-day-injured TA muscle cross-sections immunostained for BrdU and Desmin. Data represent mean±s.e.m. (n=5 WT,n=5 KO). Two-tailed unpaired Student’st-test, *Pvalue <0.05. (d) Fibrosis quantification of GA muscle cross-sections 5 days after injury. The fibrotic index represents the percentage of the injury area occupied by connective tissue. Data represent mean±s.e.m. (n=4 WT andn=4 KO). Two-tailed unpaired Student’st-test, *Pvalue <0.05. (e) Representative micrograph of perilipin immunostaining on 5-day-cardiotoxin-injured GA muscle cross-section. Scale bar represents 50 μm. (f,g) Adipocyte numbers (perilipin-positive cells) per injured (f) or un-injured (g) area from WT andOtKO mice. Data represent mean±s.e.m. (n=3 WT andn=5 KO). Two-tailed unpaired Student’st-test, NS: not significant. Figure 6: Impaired muscle regeneration in mice lacking oxytocin. ( a ) H&E (top) and eMyHC (bottom) of cardiotoxin-injured gastrocnemius (GA) muscle cross-sections from 12-month-old WT and Ot KO mice. Scale bars represent 50 μm. ( b ) Muscle regeneration quantification of 3- and 12-month-old WT or Ot KO mice was performed by scoring the number of newly formed fibres (eMyHC-positive fibres with centrally located nuclei) in the injured area of GA cross-sections. Data represent mean±s.e.m. ( n =6 WT and n =4 KO for the 3-month-old mice, n =4 WT and n =5 KO for the 12-month-old). Two-way ANOVA with post hoc Bonferroni test, * P value <0.05, NS: not significant. ( c ) Quantification of the percentage of proliferating myogenic cells (Desmin+ and BrdU+) of 3-day-injured TA muscle cross-sections immunostained for BrdU and Desmin. Data represent mean±s.e.m. ( n =5 WT, n =5 KO). Two-tailed unpaired Student’s t -test, * P value <0.05. ( d ) Fibrosis quantification of GA muscle cross-sections 5 days after injury. The fibrotic index represents the percentage of the injury area occupied by connective tissue. Data represent mean±s.e.m. ( n =4 WT and n =4 KO). Two-tailed unpaired Student’s t -test, * P value <0.05. ( e ) Representative micrograph of perilipin immunostaining on 5-day-cardiotoxin-injured GA muscle cross-section. Scale bar represents 50 μm. ( f , g ) Adipocyte numbers (perilipin-positive cells) per injured ( f ) or un-injured ( g ) area from WT and Ot KO mice. Data represent mean±s.e.m. ( n =3 WT and n =5 KO). Two-tailed unpaired Student’s t -test, NS: not significant. Full size image Moreover, similarly to 24-month-old C57/BL6 old mice, 12-month-old Ot KO mice display prematurely increased fibrosis when compared with age-matched WT littermates ( Fig. 6d , Supplementary Fig. 1b ). Appearance of adipocytes within the injured area has been reported to occur after muscle injury [36] , [37] , [38] , [39] . The number of adipocytes within the recently regenerated or un-injured muscle (assayed by perilipin staining) was generally low and a nonsignificant increase was observed in Ot KO mice, as compared with WT animals ( Fig. 6e–g ). However, we observed a clear increase in perimuscular and intermuscular adipose tissue deposition around the hind limb muscles in Ot KO versus WT littermates ( Fig. 7a ), consistent with the overall adipose tissue mass increase [17] . 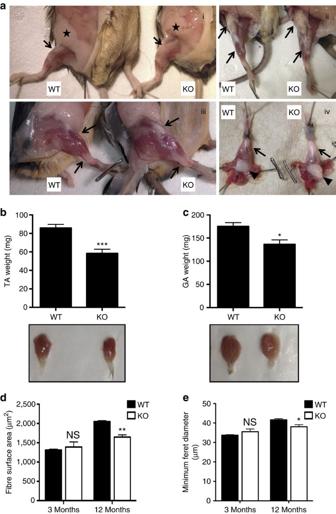Figure 7: Mice lacking oxytocin develop premature sarcopenia. (a) Representative photographs ofOtKO and WT mice hind limb skeletal muscles (right leg) after the skin was carefully removed (WT and KO mice are presented side by side on each photograph). Visualization of perimuscular adipose tissue deposition (arrows) and of exposed intermuscular adipose tissue (arrowheads). (i) Ventral view, arrows indicate the adipose tissue on the internal part of the quadriceps. The star shows thatOtKO mice display increased posterior subcutaneous adipose tissue. (ii) Ventral view showing adipose tissue deposition over the quadriceps (top arrows) and the tibialis anterior (TA) (bottom arrows). (iii) Lateral view showing adipose tissue deposition covering the quadriceps (top arrows) and the TA and gastrocnemius (GA) (bottom arrows). (iv) Dorsal view showing the intermuscular adipose tissue deposition of the hind leg (arrowheads) and the adipose tissue covering the GA muscle (arrows). As compared with the WT littermates, the KO mice have an increase in fat tissue in all the studied muscle groups, and visibly reduced muscle, which is studied in more detail and quantified below. (b) TA and (c) GA muscles from 12-month-old WT orOtKO mice were weighed. Data represent mean±s.e.m. (top), representative pictures (bottom). Two-tailed unpaired Student’st-test, *Pvalue <0.05, ***Pvalue <0.001,n=5 WT andn=10 KO mice. (d) The surface area and (e) the minimum Feret’s diameter were measured using WT andOtKO muscle cross-section stained with H&E. Data represent mean±s.e.m. (n=4 mice per group), two-way ANOVA withpost hocBonferroni test, *Pvalue <0.05, **Pvalue <0.01, NS: not significant. Figure 7: Mice lacking oxytocin develop premature sarcopenia. ( a ) Representative photographs of Ot KO and WT mice hind limb skeletal muscles (right leg) after the skin was carefully removed (WT and KO mice are presented side by side on each photograph). Visualization of perimuscular adipose tissue deposition (arrows) and of exposed intermuscular adipose tissue (arrowheads). (i) Ventral view, arrows indicate the adipose tissue on the internal part of the quadriceps. The star shows that Ot KO mice display increased posterior subcutaneous adipose tissue. (ii) Ventral view showing adipose tissue deposition over the quadriceps (top arrows) and the tibialis anterior (TA) (bottom arrows). (iii) Lateral view showing adipose tissue deposition covering the quadriceps (top arrows) and the TA and gastrocnemius (GA) (bottom arrows). (iv) Dorsal view showing the intermuscular adipose tissue deposition of the hind leg (arrowheads) and the adipose tissue covering the GA muscle (arrows). As compared with the WT littermates, the KO mice have an increase in fat tissue in all the studied muscle groups, and visibly reduced muscle, which is studied in more detail and quantified below. ( b ) TA and ( c ) GA muscles from 12-month-old WT or Ot KO mice were weighed. Data represent mean±s.e.m. (top), representative pictures (bottom). Two-tailed unpaired Student’s t -test, * P value <0.05, *** P value <0.001, n =5 WT and n =10 KO mice. ( d ) The surface area and ( e ) the minimum Feret’s diameter were measured using WT and Ot KO muscle cross-section stained with H&E. Data represent mean±s.e.m. ( n =4 mice per group), two-way ANOVA with post hoc Bonferroni test, * P value <0.05, ** P value <0.01, NS: not significant. Full size image Muscle ageing is characterized by a deficiency in muscle regeneration after injury but, most importantly, by muscle atrophy and altered muscle function observed in older individuals and defined as sarcopenia [1] , [2] . Having demonstrated that a lack of OT resulted in the diminished regeneration of old muscle after injury we next sought to examine whether OT was involved in age-associated sarcopenia. To test this hypothesis, we assessed the mass of the gastrocnemius (GA) and the TA muscles of 12-month-old Ot KO mice and their WT littermates. As shown in Fig. 7b,c , Ot deficiency resulted in significantly smaller muscles: Ot KO mice displayed a 32% decrease in muscle mass for the TA and a 22% decrease for GA as compared with their WT littermates. We further compared the muscle histology of Ot KO versus WT mice by measuring muscle fibre surface area as well as the minimum Feret diameter of muscle cross-section. Remarkably, there was a significant decrease in both the surface area and the minimum Feret diameter in Ot KO as compared with WT mice ( Fig. 7d,e ). Importantly, no difference was observed in the fibre surface area or in the minimum Feret diameter between WT and Ot KO mice when compared at 3 months of age, demonstrating that the muscle atrophy observed in Ot -deficient mice at 12 months of age was not a consequence of a developmental defect ( Fig. 7d,e ). These data demonstrate that the KO in Ot is the first known genetic defect that results in premature sarcopenia and suggest that in the absence of OT, the non-significant but noticeable decline in muscle regeneration observed at 3 months of age might contribute to the decline in muscle fibre size and increased fibrosis and fat deposition by 12 months of age ( Fig. 6b ). The role of OT in tissue homeostasis and regeneration is poorly documented and age-specific OT studies are lacking. The present work is the first to demonstrate that OT supports productive repair and maintenance of the skeletal muscle, and that age-imposed decline in OT contributes to sarcopenia. Moreover, we show that OT acts directly on muscle stem cells ( in vitro and in vivo ) and that pro-myogenic effects of OT are mediated by MAPK/ERK signalling. The age-specific decrease in OT receptor levels in muscle stem cells compounds the decline of OT itself but, importantly, significant OT receptor levels still remain in the old cells, allowing for an enhancement of myogenesis by ectopic OT. Interestingly, these findings are a mirror image of the age-imposed deregulation of TGF-β/pSmad3 signalling in muscle stem cells, where with age there is an upregulation of TGF-β1 and simultaneous elevation of the TGF-β receptor [24] , [40] . The concordant deregulation of receptors in muscle stem cells (and perhaps in tissue stem cells in general), and of the specific ligands (locally and/or in circulation) might be an interesting commonality of the ageing process. The conclusion of a pivotal role of OT in the age-specific regulation of myogenesis is emphasized by the agreement between pharmacological and genetic studies. Even though Ot KO mice could have developed compensations for the lack of OT and the high levels of myogenic IGF1, GH and so on factors that are present in these animals at a young age there is already a tendency towards a decline in muscle-regenerative capacity in Ot KO mice at 3 months of age. Such a decline is clearly manifested upon an acute administration of OT antagonist to young C57/BL6 animals. Prolong constant attenuation of muscle regeneration might contribute to premature decrease in muscle tissue health, which we observe by 1 year in Ot KO mice. While OT is a multifunctional hormone and future comprehensive work is needed in order to uncover its many age-specific effects on cells and tissues, this study strongly suggests that the lack of OT causes decline in myogenic responses of satellite cells, leading to an abandonment of muscle tissue maintenance. Considering that during normal ageing ubiquitin–proteasome proteolysis does not seem to cause the age-related muscle atrophy and that, in contrast, muscle hypertrophy and healthy functionality cannot be sustained without effective tissue remodelling [41] , [42] , [43] , the contribution of the age-specific decline in OT to the lack of myogenicity is a significant factor in muscle ageing. Importantly, no deterioration of muscle tissue or decrease in myofibre size have been detected in the 3-month-old Ot KO mice, suggesting that the genetic lack of Ot does not cause a developmental defect, and instead specifically exacerbates sarcopenia. To date, no effective treatment is available to treat or prevent sarcopenia and the primary recommendation remains exercise. Our work suggests that OT represents a physiological systemically present inducer of satellite cell activation/proliferation and hence, that systemic delivery of OT can counteract the defects in regeneration and maintenance of old muscle, which develop in part due to the age-specific decline in this hormone. Our results demonstrate that OT is one of the key age-specific systemic regulators of muscle maintenance and repair; however, it is unlikely that only one circulating molecule accounts for systemic ageing or rejuvenation and other cell fate regulatory pathways have been shown to participate in these phenomena [5] , [24] . While other strategies such as long-term activation of the Notch signalling pathway or downregulation of the TGF-β/pSmad and Wnt signalling pathways have been shown to be successful in acute rejuvenation of myogenesis [4] , [5] , [24] they come with side effects such as oncogenic transformations, inadequate haematopoiesis, broad immune deregulation and so on. Therefore, therapeutic modulation of key regulatory pathways is not an easy task. In contrast, OT is a naturally produced endocrine peptide that has little to no known detrimental side effects. Diminished circulating levels of OT are associated with pathological states such as autism in children [44] , [45] , osteoporosis [46] and depression [47] . OT is approved for use in women during parturition has been tested to improve psychological well-being in the elderly [48] and is in clinical trials to treat autism, schizophrenia and depression. Owing to its size and structure, OT can be administered easily and by multiple routes such as by intranasal inhalation. The potent positive effects of OT on muscle tissue homeostasis and repair that were uncovered in this study are thus promising for developing an effective and safe new clinical strategy where OT and OTR agonists might be potentially used as systemically applicable and sustainable molecules for combating the deterioration of muscle mass, strength and agility in the elderly. Plasma preparation and OT quantification Whole blood was collected into a citrate-treated tube and spun at 700 g for 15 min to remove cells. Supernatant was transferred to a second citrate-treated tube, spun at 1,500 g for 20 min to remove platelets. Plasma was aliquoted and stored at −80 °C. Plasma OT concentration was measured using an Enzyme Immunoassay kit (Bachem, S-1355) according to the manufacturer’s recommendation. Animals Eight-week-old male C57BL/6 mice and B6;129S-Oxttm1Wsy/J mice were purchased from the Jackson Laboratory. Twenty-two-month-old male C57BL/6 mice were purchased from the National Institute on ageing. Animals were housed and B6;129S-Oxttm1Wsy/J mice were bred at the Northwest Animal Facility (University of California, Berkeley). All procedures were performed in accordance with the administrative panel of the Office of Laboratory Animal Care, UC Berkeley. Sample size for each experiment was determined based on previously published differences between control young versus old animals in order to have sufficient statistical power, using the minimum necessary number of mice. The protocol was approved by the UC Berkeley Animal Care and Use Committee. Mice were anaesthetised by isoflurane drop and euthanized by cervical dislocation; blood samples were collected by heart puncture. Mice were injected daily with 50 μl of OT (1 μg g −1 of mice), OTA (2 μg g −1 of mice) or vehicle (HBSS) by interscapular subcutaneous injections. Satellite cell preparation and cell culture TA and GA muscles of mice were injected with a total of 10 μg of cardiotoxin (Sigma-Aldrich) per leg dissolved in phosphate-buffered saline (PBS) or were left uninjured. Muscles were dissected 3 days post injury and satellite cells were derived as previously described [4] , [24] , [25] . Briefly, harvested muscles underwent enzymatic digestion in DMEM (Mediatech) containing collagenase type II (250 U ml −1 ; Sigma-Aldrich), 10 mM HEPES and penicillin/streptomycin antibiotics (500 IU ml −1 , 0.1 mg ml −1 ; MP Biomedicals) at 37 °C for 1 h under agitation. Fat pads and tendons were removed after a quick wash with PBS and repeated rounds of muscle trituration and sedimentation were performed to purify myofibres. Myofibres were either plated or incubated with collagenase type II (40 U ml −1 , Sigma-Aldrich) and dispase (2 U ml −1 ; Invitrogen) diluted in Ham’s F-10 (Mediatech), supplemented with 10% horse serum, and penicillin/streptomycin at 37 °C for 1 h and 30 min under agitation. Suspensions were vortexed for 1 min to release satellite cells from digested fibres, passed through a 40 μm cell strainer (BD Biosciences) and pre-plated on uncoated dishes for 20 min at 37 °C, 5% CO 2 . Cells that did not adhere during pre-plating were collected and plated on Matrigel-coated (BD Biosciences) CC2-treated chamber slides (LabTek II, Thermo Fisher Scientific) in DMEM supplemented with 10% sera from the mouse they came from. Myofibres were plated in Opti-MEM (Gibco) supplemented with 10% sera from the mouse they came from for 24 h. Myofibres were then washed away and cells were either fixed for staining or induced to differentiate in the presence of DMEM 2% horse sera for 48 h. Primary myogenic progenitors were cultured in growth medium composed of Ham’s F-10 (Mediatech), penicillin/streptomycin antibiotics (500 IU ml −1 , 0.1 mg ml −1 ; MP Biomedicals) and 20% Bovine Growth Serum (Life Technologies/Hyclone), supplemented with FGF-2 (6 ng ml −1 ). To monitor the effect of OT on primary myogenic progenitor cell proliferation, cells were cultured in growth medium supplemented with OT (30 nM) alone or in combination with UO126 MEK inhibitor (10 μM). For ERK1/2 phosphorylation kinetics, primary myogenic progenitors were starved for 16 h in Opti-MEM (Gibco) before stimulation with OT (30 nM) alone or in combination with UO126 MEK inhibitor (10 μM) for 5, 10, 15 and 20 min. Western blotting Cells were lysed in RIPA buffer containing a protease inhibitor cocktail (Complete, Roche), phenylmethyl sulphonyl fluoride, NaF, β-glycerophosphate and activated sodium orthovanadate. Whole muscles were lysed in the same buffer using gentleMACS Dissociators (Miltenyi Biotec) in combination with M Tubes to homogenize the tissue. Thirty micrograms of total protein extract were resolved in Laemmli buffer by SDS–PAGE on pre-cast gels (Bio-Rad) and transferred to polyvinylidene fluoride membranes. Membranes were blocked for 30 min in 5% non-fat milk in TBS-0.05% Tween buffer. Primary antibodies against pERK1/2 (1:1,000), total ERK1/2 (1:1,000), pax7 (1:250), MHC (1:200), OTR (1:2,000) and β-Actin (1:1,000) were diluted in 5% non-fat milk in TBS-0.05% Tween buffer. Polyvinylidene fluoride membranes were incubated in antibody solutions overnight at 4 °C. Horseradish peroxidase-conjugated secondary antibodies were diluted 1:4,000 in 5% non-fat milk in TBS-0.05% Tween buffer and membranes were incubated for 2 h at room temperature. Blots were subsequently developed using Amersham ECL Plus (GE Healthcare) and analysed with a Bio-Rad Gel Doc/Chemi Doc Imageing System. Quantifications were carried out using Image J. RNA isolation and real-time RT–PCR RNA isolation was performed using an RNAeasy Mini Kit (Qiagen) according to the manufacturer’s recommendations. Reverse transcription (RT) was performed using SuperScript III First-Strand Synthesis System (Invitrogen). Real-time–PCR was performed with Bio-Rad iQ5 real-time–PCR. Primers used are as follows: GAPDH-F 5′-CCACTTGAAGGGTGGAGCCA-3′; GAPDH-R 5′-TCATGGATGACCTTGGCCAG-3′; p21-F 5′-GCCCGAGAACGGTGGAACTT-3′; p21-R 5′-GACAAGGCCACGTGGTCCTC-3′. Muscle histology We used an injury model consisting of a focal injection of cardiotoxin in the GA or the TA muscle. Muscles were dissected 3 or 5 days post injury and placed in 25% sucrose in PBS at 4 °C for 4 h. Muscle samples were then quickly rinsed and frozen in Tissue-Tek OCT for cryosectioning. Cross-sections (10 μm) were stained with Haematoxylin and Eosin or Richard-Allan Scientific Gomori trichrome (Thermo Scientific) for histology analysis. Immunocytochemistry Cells or muscle sections were fixed for 20 min in 4% paraformaldehyde, permeabilized with 0.25% Triton-X-100 in staining buffer (0.1% sodium azide and 1% bovine growth serum in PBS) for 15 min and incubated with primary antibody diluted in staining buffer overnight at 4 °C. Primary antibodies were diluted as following: BrdU: 1:200; Desmin: 1:200; Dystrophin: 1:200; eMyHC: 1:200; Ki67: 1:200; Myf5: 1:100; OTR: 1:100; Pax7: 1:20; Perilipin: 1:250. Cells or muscle sections were washed with staining buffer and incubated with an Alexa-Fluor-conjugated secondary antibody (1:2,000, Invitrogen) in staining buffer for 2 h at room temperature, washed with staining buffer and the slides were mounted with ProLong Gold antifade reagent with DAPI (P36935, Invitrogen). An additional incubation with HCl 2.5 M for 30 min was performed before the permeabilization step when cells were stained for BrdU. Chemicals and antibodies OTA desGly-NH 2 -d(CH 2 ) 5 [D-Tyr 2 ,Thr 4 ]OVT is a potent OT-selective antagonist kindly provided by Professor Maurice Manning from the University of Toledo [49] , [50] . OT was purchased from Bachem (H-2510). MEK inhibitor UO126 was purchased from Cell Signalling (9903) and PD98059 from Tocris (1213). Antibodies against eMyHC (F1.652) and Pax7 were purchased from the Developmental Studies Hybridoma Bank. Anti-OTR antibody was purchased from Proteintech (23045-1-AP). Antibodies against Desmin (ab15200), Ki67 (ab15580), BrdU (ab6326) and Dystrophin (ab3149) were purchased from Abcam. Antibodies against Phospho-p44/42 MAPK (ERK1/2) (Thr202/Tyr204) and p44/42 MAPK (ERK1/2) and β-Actin were purchased from Cell Signalling (4370, 4696 and 4967, respectively). Anti-Perilipin A/B antibody was purchased from Sigma-Aldrich (P1873) and antibodies against Myf5 and MHC were purchased from Santa Cruz Biotechnology (SC-302 and SC-20641, respectively). Fluorophore-conjugated secondary antibodies (Alexa Fluor) were purchased from Invitrogen. horseradish peroxidase-conjugated secondary antibodies were purchased from Santa Cruz Biotechnology. Fibre size Fibre surface area and Feret minimum diameter were measured using the Image J software on haematoxylin and eosin-stained muscle cross-sections. Fibrosis quantification Fibrosis was quantified as previously described [5] . Briefly, GA muscle cross-sections were immunostained for eMyHC. The total injured area and the fibre area of all eMyHC-positive fibres were measured using the Image J software. The ‘Fibrotic Index’ was calculated as: (1−(total eMyHC+fibres area/total injury area)) × 100%. How to cite this article: Elabd, C. et al. Oxytocin is an age-specific circulating hormone that is necessary for muscle maintenance and regeneration. Nat. Commun. 5:4082 doi: 10.1038/ncomms5082 (2014).